IM30 triggers membrane fusion in cyanobacteria and chloroplasts The thylakoid membrane of chloroplasts and cyanobacteria is a unique internal membrane system harbouring the complexes of the photosynthetic electron transfer chain. Despite their apparent importance, little is known about the biogenesis and maintenance of thylakoid membranes. Although membrane fusion events are essential for the formation of thylakoid membranes, proteins involved in membrane fusion have yet to be identified in photosynthetic cells or organelles. Here we show that IM30, a conserved chloroplast and cyanobacterial protein of approximately 30 kDa binds as an oligomeric ring in a well-defined geometry specifically to membranes containing anionic lipids. Triggered by Mg 2+ , membrane binding causes destabilization and eventually results in membrane fusion. We propose that IM30 establishes contacts between internal membrane sites and promotes fusion to enable regulated exchange of proteins and/or lipids in cyanobacteria and chloroplasts. Engulfment of an early photosynthetic cyanobacterium by a non-photosynthetic cell resulted in the evolution of present chloroplasts, the plant-specific cell organelles where photosynthesis takes place. Both chloroplasts and cyanobacteria contain two internal membranes: the inner envelope (IE) in chloroplasts, which corresponds to the cyanobacterial cytoplasmic membrane (CM), as well as the thylakoid membrane (TM), a unique internal membrane system harbouring the complexes of the photosynthetic electron transfer chain. Despite their apparent importance, remarkably little is known about the biogenesis and maintenance of TMs. Processes involved in TM biogenesis, such as protein, lipid and pigment synthesis, as well as their processing, transport and assembly, have to be controlled and aligned to finally assemble this complex membrane system. Vesicle fission at the IE and vesicle fusion have been implicated in the de novo formation of the TM network in greening chloroplasts [1] , [2] . Synthesis of galactolipids, important TM building blocks, is localized within the chloroplast IE membrane [3] , and thus a mechanism ensuring continuous transport to the TM must exist. In cyanobacteria, the biogenesis of certain membrane proteins appears to commence within the cyanobacterial CM but continues in the TM [4] , [5] , and thus here too a transfer mechanism must exist. Regulated material transfer between the IE/CM and the TMs have been proposed to be mediated by vesicular transport or via direct connections between the membrane systems [6] , [7] . Direct connections between the IE and TM have been observed in chloroplasts [8] , [9] , and TM membrane reorganization is also suggested to involve dynamic fission and fusion events, as found in the membranes of the mitochondria, endoplasmic reticulum and the Golgi apparatus [10] . In the cyanobacterium Synechocystis sp. PCC 6803, direct connections between the CM and TM have also been observed [11] . Thus, despite the lack of definitive proof, the existence of direct membrane connections in chloroplasts and cyanobacteria cannot be simply dismissed. Whereas in cold-adapted chloroplasts vesicles appeared, which resemble COPII vesicles found in the cytosol [1] , [12] , [13] , the existence of vesicles in cyanobacteria remains the subject of debate [14] . However, in recent bioinformatics analyses, chloroplast-localized components of a vesicular transfer system have been identified, and some of the identified proteins are also conserved in cyanobacteria [15] , [16] . Thus, several recent observations indicate that vesicular transfer processes are potentially involved in TM biogenesis and maintenance. It should be noted that both direct membrane fusion and vesicle transfer likely involve proteins, which mediate membrane fusion. Although fusion proteins have been well characterized for the exocytotic pathway in eukaryotes (for example, SNARE proteins) [17] and viral entry mechanisms [18] , a protein-triggering membrane fusion in chloroplasts and/or cyanobacteria has yet to be identified. Interestingly, depletion of the protein IM30, a ∼ 30-kDa protein conserved in chloroplast and cyanobacteria, results in a significant reduction of TMs and loss of cell viability in both chloroplasts and cyanobacteria [19] , [20] , [21] , indicating the involvement of IM30 in TM biogenesis and/or maintenance. Despite the lack of a transmembrane domain, IM30 has been suggested to interact with membranes, initially based on the observation that IM30 is in close proximity to membranes in immuno-gold analyses and its co-sedimentation with membranes during ultracentrifugation [21] , [22] , [23] , [24] . However, given that IM30 forms oligomeric structures, with molecular masses exceeding 2 MDa (ref. 25 ), these protein structures will trivially co-sediment with membranes. The closely related phage shock protein A (PspA) of Escherichia coli has been demonstrated to bind to the negatively charged lipid phosphatidylglycerol (PG) [26] , and thus IM30 binding to the negatively charged PG appears to be likely [27] . Mainly based on analyses of IM30-depleted chloroplasts and cyanobacteria, diverse functions have been suggested for IM30. An Arabidopsis thaliana mutant lacking IM30 was not only defective in TM biogenesis but cold-induced vesicles were also no longer observed at the IE, indicating involvement of the protein in vesicle formation [19] . Consequently, the name ‘vesicle-inducing protein in plastids 1’ (Vipp1) has been suggested. However, further studies have indicated that IM30 is involved in maintaining the structure and stability of internal membranes in chloroplasts and cyanobacteria, similar to its bacterial homologue PspA, and thus has a more protective function [27] , [28] . In addition, IM30 has been found to enhance protein translocation via the chloroplast Tat pathway [29] and involvement in photosystem biogenesis has been suggested [21] , [30] , [31] , [32] . Currently, no model combining these diverse IM30 functions has been proposed, and the exact role of IM30 remains enigmatic. Here we show that IM30 binds as an oligomeric ring in a well-defined geometry specifically to membranes containing anionic lipids. Triggered by Mg 2+ , membrane binding eventually results in membrane fusion, and IM30-established membrane contacts and fusion eventually allow dynamic remodelling of TM liposomes, which we propose may permit regulated exchange of proteins and/or lipids between internal membranes in cyanobacteria and chloroplasts. IM30 binds to the negatively charged TM lipids PG and SQDG As the exact mode of IM30 binding to membranes still is unknown, we first investigated the co-localization of IM30 with TMs more dependably by sucrose density (SD) gradient centrifugation ( Fig. 1a ). Although the IM30 oligomers were found in the pellet fraction, a significant portion of the protein co-localized with TMs, pointing to a direct interaction of IM30 with cyanobacterial membranes. Similarly, heterologously produced IM30 ( Supplementary Fig. 1 ) co-migrated consistently with urea-washed TMs ( Fig. 1b ), whereas in the absence of TMs, IM30 was found exclusively in the pellet fraction ( Fig. 1c ). Clearly, the membrane-binding properties are preserved in the recombinant IM30, so that the IM30-binding affinity to liposomes with different lipid compositions could be readily determined, using this purified IM30. 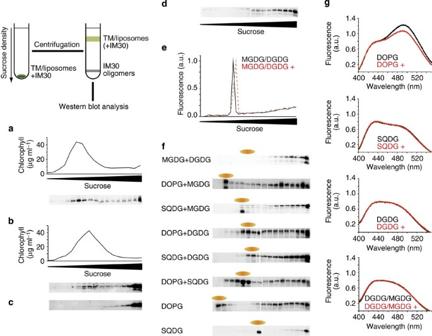Figure 1: IM30 interaction with membrane lipids. SD gradient flotation analysis of (a) native IM30 attached toSynechocystismembranes, (b) heterologously expressed IM30 added to urea-washed membranes and (c) solely heterologously expressed IM30. Samples were separated on 34–68% SD gradients, fractionated and analysed by SDS–PAGE and western blot analyses, using an anti-IM30 antibody. Localization of the membranes within the gradient was determined by monitoring chlorophyll absorption (shown on top of the western blot ina,b). (d–f) Liposomes mixed with IM30 (e,f) as well as solely IM30 (d) were separated on a 5–50% SD gradient prior to analysis. The fluorescent probe C6-NBD-PE was incorporated into the liposomes (1:500) for detection, and the position of the liposomes within the gradient was determined by fluorescence spectroscopy. The localization of the liposomes is shown for MGDG/DGDG-containing liposomes and thereafter only indicated above each western blot. The analyses were repeated three times and representative western blots are shown. Full scans of western blots are shown inSupplementary Fig. 8. (g) Peripheral binding of IM30 to liposomes was additionally followed by monitoring changes in the Laurdan fluorescence emission after excitation at 350 nm. Normalized fluorescence emission spectra are shown in the absence (black) and presence of 2.5 μM IM30 (red). Decreased fluorescence emission at 490 nm, that is, increased lipid acyl chain order, indicates peripheral binding of IM30. The experiment was performed four times. See alsoSupplementary Fig. 2. Figure 1: IM30 interaction with membrane lipids. SD gradient flotation analysis of ( a ) native IM30 attached to Synechocystis membranes, ( b ) heterologously expressed IM30 added to urea-washed membranes and ( c ) solely heterologously expressed IM30. Samples were separated on 34–68% SD gradients, fractionated and analysed by SDS–PAGE and western blot analyses, using an anti-IM30 antibody. Localization of the membranes within the gradient was determined by monitoring chlorophyll absorption (shown on top of the western blot in a , b ). ( d – f ) Liposomes mixed with IM30 ( e , f ) as well as solely IM30 ( d ) were separated on a 5–50% SD gradient prior to analysis. The fluorescent probe C6-NBD-PE was incorporated into the liposomes (1:500) for detection, and the position of the liposomes within the gradient was determined by fluorescence spectroscopy. The localization of the liposomes is shown for MGDG/DGDG-containing liposomes and thereafter only indicated above each western blot. The analyses were repeated three times and representative western blots are shown. Full scans of western blots are shown in Supplementary Fig. 8 . ( g ) Peripheral binding of IM30 to liposomes was additionally followed by monitoring changes in the Laurdan fluorescence emission after excitation at 350 nm. Normalized fluorescence emission spectra are shown in the absence (black) and presence of 2.5 μM IM30 (red). Decreased fluorescence emission at 490 nm, that is, increased lipid acyl chain order, indicates peripheral binding of IM30. The experiment was performed four times. See also Supplementary Fig. 2 . Full size image Binding of IM30 to model membranes derived from natural TM lipids was analysed by centrifugation on 5–50% SD gradients. The fluorescent probe [(2S)-3-[2-aminoethoxy(hydroxy)phosphoryl]oxy-2-[6-[(4-nitro-2,1,3-benzoxadiazol-7-yl)amino]hexanoyloxy]propyl] hexadecanoate (C6-NBD-PE) was always incorporated into the liposomes, to allow optical detection of the liposomes. The main TM lipids are the uncharged galactolipids monogalactosyldiacylglycerol (MGDG) and digalactosyldiacylglycerol (DGDG), which account for 50–60% and ∼ 20% of the lipids, respectively, whereas the two negatively charged lipids sulfoquinovosyldiacylglycerol (SQDG, ∼ 12%) and PG ( ∼ 8%) constitute minor fractions [33] , [34] , [35] . IM30 alone localized within the lower half of this SD gradient, mainly pelleting, because of its propensity to form high-molecular-mass oligomers ( Fig. 1d ). However, a fraction of the protein consistently co-localizes with liposomes, containing either solely the anionic lipids SQDG and PG or a combination of neutral and anionic lipids ( Fig. 1e, f ). In contrast, co-localization of IM30 with liposomes composed of the two neutral galactolipids MGDG and DGDG was not observed. Thus, IM30 interaction with membranes appears to be mediated by the anionic lipids PG and SQDG. To further elucidate whether co-localization with membranes was caused by a direct membrane interaction, we investigated interaction of IM30 with liposomes by using the fluorescent probe Laurdan, which monitors changes in the membrane lipid order, for example, caused by peripheral binding of a protein ( Fig. 1g ). The decrease of the Laurdan fluorescence emission at 490 nm indicates that IM30 affects the lipid order by binding to pure PG membranes. In contrast, addition of IM30 did not significantly influence the Laurdan signal monitored in pure SQDG membranes, probably due to the fact that the acyl chain order is already high in SQDG membranes, and binding of IM30 might therefore not induce a further decrease in the 490-nm emission. Nevertheless, when using another (non-physiological) neutral lipid as a background, interaction of IM30 with both, PG- and SQDG-containing membranes, was again observed, but not with MGDG- or DGDG-containing membranes ( Supplementary Fig. 2 ). Together, the SD-gradient and Laurdan experiments strongly indicate that IM30 directly interacts with negatively charged TM lipids, and that membrane-bound IM30 remodels the membrane structure. IM30 affects the membrane order and promotes liposome fusion As peripheral binding of IM30 to membrane surfaces is expected to affect surface properties, we monitored liposome–liposome interactions in the absence and presence of IM30, with increasing concentrations of Na + , K + , Ca 2+ or Mg 2+ ( Fig. 2a ). Divalent cations severely affect galactolipid-containing liposomes and are known to induce liposome aggregation [36] , [37] . As expected, addition of increasing Ca 2+ and Mg 2+ concentrations resulted in liposome aggregation, starting at 6 and 17.5 mM, respectively. Although addition of IM30 alone had no visible effect, the simultaneous addition of IM30 and Ca 2+ or Mg 2+ caused interactions to start at significantly lower ion concentrations. However, Mg 2+ -induced liposome contacts differed dramatically in the presence of IM30, as the scattering signal decreased at further increasing Mg 2+ concentrations until it levelled off. In contrast, Na + and K + had no significant effect on liposome aggregation. Together, these results indicate that IM30 functionally cooperates with Mg 2+ at membranes. However, liposome aggregation could simply reflect liposome–liposome contacts but could also indicate liposome fusion. 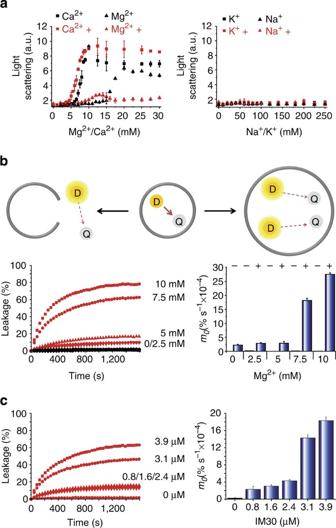Figure 2: IM30 influences MGDG/PG liposome aggregation induced by divalent cations. (a) MGDG/PG (60:40) liposome aggregation determined in the presence or absence of IM30 and increasing Ca2+and Mg2+(left) or Na+and K+(right) concentrations. Error bars: s.d. (N=4). (b) Dye-loaded MGDG/PG (60:40) liposomes were mixed with 3.9 μM IM30 and increasing Mg2+concentrations as indicated, and the increase in ANTS fluorescence emission due to content release or vesicle fusion was monitored over 1,600 s (left). Inc, fluorescence emission was monitored after mixing liposomes with 7.5 mM Mg2+and increasing IM30 concentrations (left). In the right panels ofbandc, the increases in fluorescence emission in the initial phases, calculated by linear regression, are shown. Error bars: s.d. (N=3). Figure 2: IM30 influences MGDG/PG liposome aggregation induced by divalent cations. ( a ) MGDG/PG (60:40) liposome aggregation determined in the presence or absence of IM30 and increasing Ca 2+ and Mg 2+ (left) or Na + and K + (right) concentrations. Error bars: s.d. ( N =4). ( b ) Dye-loaded MGDG/PG (60:40) liposomes were mixed with 3.9 μM IM30 and increasing Mg 2+ concentrations as indicated, and the increase in ANTS fluorescence emission due to content release or vesicle fusion was monitored over 1,600 s (left). In c , fluorescence emission was monitored after mixing liposomes with 7.5 mM Mg 2+ and increasing IM30 concentrations (left). In the right panels of b and c , the increases in fluorescence emission in the initial phases, calculated by linear regression, are shown. Error bars: s.d. ( N =3). Full size image To further probe the impact of IM30 on the membrane structure and stability, we next monitored the release of soluble liposome content upon IM30 addition ( Fig. 2b ). Adding only IM30 to MGDG/PG liposomes loaded with a fluorophore/quencher pair without the addition of ions resulted in membrane binding, but did not significantly destabilize the membrane. Furthermore, over a concentration range of 0–10 mM, the addition of solely Mg 2+ also did not induce liposome leakage. However, the addition of increasing Mg 2+ concentrations to IM30-containing liposomes resulted in an increased destabilization of the membrane and in liposome content release. The observed leakage rates strongly depend on both Mg 2+ and protein concentrations ( Fig. 2b,c ). Clearly, IM30 and Mg 2+ destabilize the vesicular membrane structure in a cooperative manner. Sum frequency generation (SFG) vibrational spectroscopy of a PG lipid monolayer further corroborates the IM30-induced perturbation of the lipid layer structure ( Supplementary Fig. 3 ) by showing that the interaction with IM30 decreases the lipid acyl chain ordering and affects the lipid orientation. In summary, the above observations show that IM30 interacts with membranes and together with Mg 2+ promotes membrane destabilization. Interaction with and the destabilization of membranes are both essential for an effective trigger of membrane fusion. Thus, to explore a potential fusogenic activity of IM30, we performed a membrane fusion assay using labelled MGDG/PG liposomes. Fusion of labelled with unlabelled liposomes resulted in an increase of the donor fluorescence ( Fig. 3 ). Neither IM30 nor Mg 2+ alone induced liposome fusion, whereas IM30-mediated membrane fusion was observed above 5 mM Mg 2+ ( Fig. 3a,b ). Higher Mg 2+ concentrations resulted in a dramatic increase of the fusion rates, and fusion efficiencies of ∼ 100% were reached at 10 mM Mg 2+ and 2.5 μM IM30. Thus, the membrane fusion activity of IM30 clearly depends on Mg 2+ . It is interesting to note that this membrane fusion activity was not observed for an IM30 mutant, which still forms the oligomeric ring structures at membrane surfaces observed for the wild-type protein ( Supplementary Fig. 4 ). 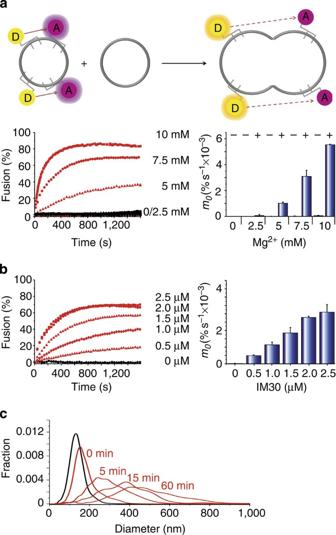Figure 3: IM30 and Mg2+-mediated vesicle fusion. (a) MGDG/PG liposomes, containing the donor and acceptor dye, were mixed with non-labelled liposomes, and the increase in donor fluorescence emission was monitored over 1,600 s after addition of 2.5 μM IM30 and increasing Mg2+concentrations (left). Inb, the liposomes were mixed with increasing IM30 concentrations in the presence of 7.5 mM Mg2+. 0 and 100% fusion rates were determined in control experiments to calculate the fusion efficiency for each sample. The right panels ofaandbshow the increases in fluorescence emission in the initial phases calculated by linear regression. Error bars: s.d. (N=3). (c) The size distribution of MGDG/PG liposomes was determined by nanoparticle tracking analysis. The liposomes prepared by extrusion had a mean diameter of 130 nm (black). Addition of Mg2+and 1.3 μM IM30 immediately slightly increased the mean diameter (red, 0 min). With increasing incubation time (red curves), the liposome size distribution shifted to larger diameters. The experiment was repeated two times. Figure 3: IM30 and Mg 2+ -mediated vesicle fusion. ( a ) MGDG/PG liposomes, containing the donor and acceptor dye, were mixed with non-labelled liposomes, and the increase in donor fluorescence emission was monitored over 1,600 s after addition of 2.5 μM IM30 and increasing Mg 2+ concentrations (left). In b , the liposomes were mixed with increasing IM30 concentrations in the presence of 7.5 mM Mg 2+ . 0 and 100% fusion rates were determined in control experiments to calculate the fusion efficiency for each sample. The right panels of a and b show the increases in fluorescence emission in the initial phases calculated by linear regression. Error bars: s.d. ( N =3). ( c ) The size distribution of MGDG/PG liposomes was determined by nanoparticle tracking analysis. The liposomes prepared by extrusion had a mean diameter of 130 nm (black). Addition of Mg 2+ and 1.3 μM IM30 immediately slightly increased the mean diameter (red, 0 min). With increasing incubation time (red curves), the liposome size distribution shifted to larger diameters. The experiment was repeated two times. Full size image IM30-triggered liposome fusion was further analysed by single-particle tracking analysis ( Fig. 3c ). Before addition of Mg 2+ and IM30, the liposomes had a mean diameter of 130 nm. Addition of Mg 2+ and 1.3 μM IM30 immediately resulted in a slight increase of the mean vesicle diameter, and with increasing incubation time, the liposome size distribution shifted to larger diameters due to liposome fusion. IM30 triggers membrane fusion by membrane destabilization Cryo-electron microscopy revealed that the diameter of the analysed MGDG/PG liposomes is typically less than 200 nm ( Fig. 4a ), in agreement with the single-particle tracking analysis. Upon addition of either IM30 or Mg 2+ , the structure of these liposomes did not change significantly ( Fig. 4b,c ). Despite the observation of loose contacts between different liposomes in the presence of IM30, strong aggregation or fusion was not visible. As depletion of IM30 in A. thaliana chloroplasts has caused decoupling of TMs and the IE [28] , IM30 potentially mediates a loose contact between neighbouring membranes. Notably, in the presence of high Mg 2+ concentrations, liposomes were essentially no longer found inside the holes of the holey carbon film, but mostly on the carbon itself. However, upon addition of IM30 and Mg 2+ , the liposomes were found in large amounts inside the holes ( Fig. 4d,e ), suggesting that attachment of IM30 affects the surface properties of the liposomes. Furthermore, the size of the liposomes had increased significantly, indicating fusion events, and extended contact surface areas between vesicles were apparent. 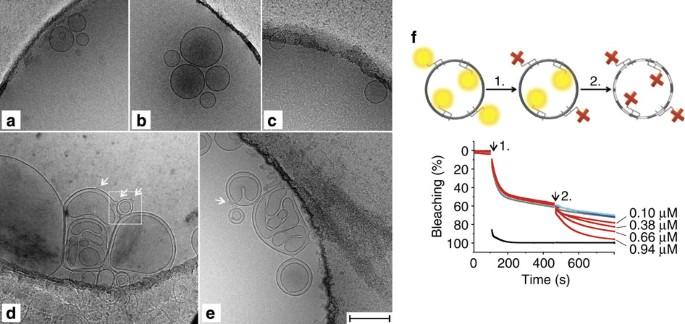Figure 4: IM30 disturbs the membrane structure and thereby triggers membrane fusion. (a–e) Cryo- transmission electron microscope images of pure MGDG/PG liposomes (a), of liposomes mixed with solely IM30 (b) or Mg2+(c), as well as of liposomes mixed with both, IM30 and Mg2+(d,e). Notably, at high Mg2+concentrations, vesicles were essentially no longer found inside the holes of the holey carbon film, but mostly on the carbon itself. In contrast, with both IM30 and Mg2+present, the vesicles were found in large amounts inside the holes (d,e), suggesting that attachment of IM30 affects the surface properties of the liposomes. Furthermore, note the large compartmentalized liposomes indande, as well as the extended connection between two liposomes ind. Arrows indicate extra electron density found at the liposome surface. The area boxed indis enlarged inFig. 5. Scale bar, 200 nm. The magnification was identical ina–e. EM micrographs were taken after 1 min incubation with Mg2+and/or IM30. (f) Sodium dithionite was added to NBD-labelled MGDG/PG liposomes (1), resulting in immediate quenching of the NBD fluorescence of the outer membrane leaflet. (2) When nothing further (light grey), solely 0.94 μM IM30 (light blue) or solely 11 mM MgCl2(dark blue) was added to the liposomes, the fluorescence did not considerably decrease further. After addition of increasing IM30 concentrations at a constant MgCl2concentration of 7.5 mM (red curves), the NBD-fluorescence decreased further in an IM30 concentration-dependent manner. Addition of Triton X-100, which dissolves the liposomal membranes, results in an immediate quenching of the entire NBD-fluorescence (black). The experiment was repeated two times. Figure 4: IM30 disturbs the membrane structure and thereby triggers membrane fusion. ( a – e ) Cryo- transmission electron microscope images of pure MGDG/PG liposomes ( a ), of liposomes mixed with solely IM30 ( b ) or Mg 2+ ( c ), as well as of liposomes mixed with both, IM30 and Mg 2+ ( d , e ). Notably, at high Mg 2+ concentrations, vesicles were essentially no longer found inside the holes of the holey carbon film, but mostly on the carbon itself. In contrast, with both IM30 and Mg 2+ present, the vesicles were found in large amounts inside the holes ( d , e ), suggesting that attachment of IM30 affects the surface properties of the liposomes. Furthermore, note the large compartmentalized liposomes in d and e , as well as the extended connection between two liposomes in d . Arrows indicate extra electron density found at the liposome surface. The area boxed in d is enlarged in Fig. 5 . Scale bar, 200 nm. The magnification was identical in a – e . EM micrographs were taken after 1 min incubation with Mg 2+ and/or IM30. ( f ) Sodium dithionite was added to NBD-labelled MGDG/PG liposomes (1), resulting in immediate quenching of the NBD fluorescence of the outer membrane leaflet. (2) When nothing further (light grey), solely 0.94 μM IM30 (light blue) or solely 11 mM MgCl 2 (dark blue) was added to the liposomes, the fluorescence did not considerably decrease further. After addition of increasing IM30 concentrations at a constant MgCl 2 concentration of 7.5 mM (red curves), the NBD-fluorescence decreased further in an IM30 concentration-dependent manner. Addition of Triton X-100, which dissolves the liposomal membranes, results in an immediate quenching of the entire NBD-fluorescence (black). The experiment was repeated two times. Full size image Thus far, the observations indicate that IM30 is surface active, perturbs the structure of lipid bilayers and induces membrane fusion. However, although membrane fusion is clearly observed, the assays presented in Figs 2 and 3 cannot distinguish between membrane fusion directly controlled by IM30 and spontaneous fusion induced by membrane destabilization. The formation of large multilamellar liposomes upon addition of IM30 and Mg 2+ , as observed by cryo-electron microscopy ( Fig. 4d,e ), indicated that IM30 is not a canonical membrane fusion protein. Liposome fusion mediated by classical membrane fusion proteins would result in unilamellar liposomes with increased size. In contrast, IM30 appears to enable membrane fusion by membrane destabilization and remodelling. To test whether liposome fusion is indeed caused by IM30-triggered membrane destabilization, we prepared liposomes labelled with NBD in both leaflets of the lipid bilayer. As shown in Fig. 4f , the addition of sodium dithionite to the liposomes selectively quenched the NBD fluorescence in the outer membrane leaflet. In contrast, the NBD probes of the inner leaflet are not quenched by sodium dithionite as the membrane is impermeable for the quencher. In contrast, when the membrane is solubilized by addition of a detergent, the fluorescence is completely quenched. Also, addition of IM30 further reduced the NBD fluorescence, indicating that the fluorescent probes located in the inner membrane leaflet were reached by the quencher. Thus, addition of IM30 disturbs the membrane structure sufficiently to allow sodium dithionite to enter the liposomes. Apparently, IM30-triggered membrane remodelling and destabilization results in spontaneous membrane fusion, which explains the formation of multilamellar liposomes. IM30 binds as a ring to lipid bilayers Throughout the samples analysed by cryo-electron microscopy, side views of areas with additional electron density at the membrane surface are visible (arrows in Fig. 4d,e ). This extra electron density matches in size and shape oligomeric IM30 rings attached to the membrane surfaces, as shown in Fig. 5a,b . To further corroborate this membrane-binding structure, the structure of IM30 bound to model MGDG/PG lipid monolayers at the air–water interface was studied using SFG vibrational spectroscopy ( Fig. 5c ). The peak near 1,740 cm −1 in the surface-specific vibrational spectra is caused by lipid carbonyls; the peak near 1,650 cm −1 by backbone amide vibrations of IM30. The large magnitude of the protein signal with respect to the lipid signal confirms stable and ordered binding of IM30 to the surface of MGDG/PG monolayers, and the 1,650 cm −1 peak position indicates a mostly helical secondary structure. The SFG-spectrum can only be reproduced by simulation with the IM30 protein monomers oriented predominantly perpendicular to the membrane surface, indicating that IM30 binds as ring structures to membrane surfaces ( Supplementary Fig. 5 ). In the transmission electron microscope images, superimposition of the extra electron density at the vesicle surface with a three-dimensional (3D) reconstruction of an IM30 ring agrees very well with the concept of perpendicular binding of rings ( Fig. 5d ). However, in case of the wild-type IM30 protein, we observed IM30 rings only in a few sparse areas of the liposome. In contrast, in case of the fusion-incompetent IM30 mutant ( Supplementary Fig. 4b ), the liposome surface is more extensively decorated with IM30 rings. This indicates that the oligomeric ring structure is destabilized and disassembles during or after liposome fusion. The role of the Mg 2+ in the binding, alignment and ring formation of IM30 at the membrane surface cannot be determined with certainty yet. However, the observed decrease (by a factor >3) of the protein SFG-response in the absence of Mg 2+ ( Supplementary Fig. 6 ) suggests that Mg 2+ is able to provide the critical membrane-protein link in the surface-binding process. 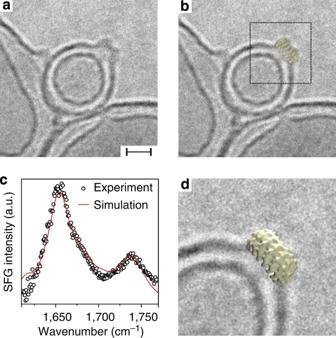Figure 5: IM30 rings bind perpendicularly to membrane surfaces. (a) Cryo-TEM image showing IM30 as extra electron density attached to a liposome. Scale bar, 20 nm. (b) Superposition of the extra density with the side-view of a 3D reconstructed IM30 ring being depicted in projection view (approximately 30 nm in diameter). (c) Experimental (circles) and calculated (line) SFG-spectra of IM30 bound to a model MGDG/PG monolayer at the air–water interface using the ssp polarization combination. The experiment was repeated two times. The calculated spectra match the experimental data well for upright monomer orientations. A tilt angle of 0° with respect to the surface normal was used for the calculation shown. (d) Magnification of the box inb, depicting the 3D reconstruction in an isosurface view. Note that the 3D reconstruction matches the extra electron density in size and shape, indicating perpendicular binding of IM30 to the membrane surface. Figure 5: IM30 rings bind perpendicularly to membrane surfaces. ( a ) Cryo-TEM image showing IM30 as extra electron density attached to a liposome. Scale bar, 20 nm. ( b ) Superposition of the extra density with the side-view of a 3D reconstructed IM30 ring being depicted in projection view (approximately 30 nm in diameter). ( c ) Experimental (circles) and calculated (line) SFG-spectra of IM30 bound to a model MGDG/PG monolayer at the air–water interface using the ssp polarization combination. The experiment was repeated two times. The calculated spectra match the experimental data well for upright monomer orientations. A tilt angle of 0° with respect to the surface normal was used for the calculation shown. ( d ) Magnification of the box in b , depicting the 3D reconstruction in an isosurface view. Note that the 3D reconstruction matches the extra electron density in size and shape, indicating perpendicular binding of IM30 to the membrane surface. Full size image Understanding membrane fusion mechanisms has been an important focus of biochemistry and biophysics research in the past years. Accordingly, proteins involved in fusion processes, such as exocytotic pathways in eukaryotes (SNARE proteins) and viral entry have received substantial interest and are the topics of increasingly dynamic fields of research. Membrane fusion typically not only requires the tethering activity of proteins but also involves significant membrane remodelling. Membrane fusion/fission processes in the endoplasmic reticulum, the Golgi apparatus or in the mitochondria involve well-defined protein machineries, which help to overcome the energy barrier associated with such processes [38] , [39] , [40] . Although it is clear that fusion proteins are essential for the formation and maintenance of TMs, surprisingly, not a single fusion-inducing protein has been identified in TM-containing organisms yet. Fusion of individual TM sheets and of the CM and TMs has previously been observed in chloroplasts and cyanobacteria [9] , [11] , and in chloroplasts, with changing light conditions the architecture of the TM network rearranges, involving membrane fission and fusion events [10] . As in chloroplasts, also in cyanobacteria, the TM network can be highly interconnected [41] , and it is thus likely that the TM system of cyanobacteria is as dynamic as in chloroplasts and undergoes remodelling under changing growth conditions or in the course of development [6] . However, proteins involved in this dynamic rearrangement of membranes in chloroplasts have not yet been identified [42] . The recent observation that in maize mesophyll cell chloroplasts, which harbour a rather extended TM network, the amount of IM30 is ∼ 10-fold higher than in maize bundle sheet chloroplasts indicates a crucial involvement of IM30 in TM biogenesis and maintenance [43] . Our results show that IM30 is indeed a potential key player for TM formation, rearrangement and maintenance in chloroplasts and cyanobacteria, by triggering membrane fusion. IM30 is clearly able to bind, assemble and manipulate TMs and thereby triggers fusion of membrane structures. A central role of IM30 in triggering membrane fusion explains the various pleiotropic functions ascribed to IM30 in the past, mainly based on studies using higher plants, algae or cyanobacteria with decreased IM30 contents. Lipid transport [24] , [44] , vesicle budding or fission [19] , protein translocation and insertion [29] , [45] , [46] , membrane modification [28] , [47] , as well as biogenesis of photosystems [21] , [30] , [48] have been ascribed to IM30. Our study now provides a unifying explanation for the observations and proposed functions: As its homologue PspA [26] , IM30 binds to negatively charged lipid bilayers and affects the membrane structure. Initiated by Mg 2+ , IM30 can mediate membrane contacts and triggers membrane fusion, and thereby enables regulated exchange of proteins and/or lipids throughout different internal membranes. After membrane attachment, the IM30 ring structures appear to disassemble on the membrane surface during or after the membrane fusion event. The observation that impaired ring disassembly, as seen in case of the IM30 mutant ( Supplementary Fig. 4 ), coincides with inhibited membrane fusion, indicates that ring disassembly is essential for initiating membrane fusion. In our in vitro system, membrane fusion is initiated by destabilization of the lipid bilayer structure resulting in spontaneous membrane fusion. However, it appears likely that additional proteins with tethering activity are involved in vivo to induce and control selective membrane fusion. These proteins might involve dynamin-related GTPases, such as FZL, or SNARE-like proteins, which have been identified in chloroplasts and cyanobacteria [15] , [16] , [49] , [50] . The notion that the IM30 fusion activity depends on Mg 2+ agrees well with the observation that Mg 2+ is generally involved in enzyme regulation within chloroplasts and cyanobacteria [51] . As IM30 is conserved in both chloroplasts and cyanobacteria, the biogenesis and maintenance of TMs may well be controlled by IM30-mediated membrane remodelling. IM30 expression and purification The Synechocystis IM30 was heterologously expressed in E. coli BL21 (DE3) cells as an N-terminally deca His-tagged protein, using the plasmid pRSET-SynVipp1 (refs 21 , 25 ). When the liquid E. coli culture had reached an OD 600 of ∼ 0.8, protein expression was induced by addition of 0.5 mM isopropyl-β-D-thiogalactopyranoside. After 4 h, cells were harvested, resuspended in buffer (300 mM NaCl, 50 mM sodium phosphate, 20 mM imidazol, pH 7.6) and broken by ultrasonification. After centrifugation (10,000 g , 4 °C, 15 min), the supernatant was loaded onto a nickel-nitrilotriacetic acid agarose column (Qiagen). The column was washed three times with buffer containing increasing imidazol concentrations (20, 50 and 100 mM), and the protein was finally eluted with buffer containing 500 mM imidazol. Before subsequent analyses, the protein was dialysed against 20 mM HEPES (pH 7.6). IM30 purity was confirmed on 14% SDS polyacrylamide gels ( Supplementary Fig. 1 ). After purification, the protein was dialysed against 20 mM Hepes-KOH, pH 7.6 (HEPES). SD gradient centrifugations SD gradients were produced and fractionated using the Gradient Station (Biocomp). For analyses, all gradients were centrifuged at 100,000 g for 6 h and immediately fractionated. Individual fractions were analysed by fluorescence spectroscopy and fractionated proteins were separated on 14% SDS–PAGE gels with subsequent immunoblot analysis, using an anti-IM30 antiserum [25] (dilution 1:1,000) and a peroxidase-coupled anti-rabbit secondary antibody (#A0545, Sigma; diluted 1:10,000). The ‘ECLTM Prime Western Blotting Detection Reagent’ (GE Healthcare) was used following the manufacturer’s instruction, to visualize the secondary antibody using a STELLA imaging system (Raytest). Membrane purification Synechocystis PCC 6803 cells were cultivated photo-mixotrophically in liquid BG11 media supplemented with 5 mM glucose [21] . Erlenmeyer flasks were incubated at 30 °C on an orbital shaker (150 r.p.m.) under fluorescent white light at a light intensity of 30 μmol photons per m 2 per s 1 (ref. 21 ). Cells were harvested in the mid-log phase ( OD 730 of ∼ 1). After cell lyses, the cell lysate was split into two fractions: one was further purified in HEPES buffer and the other one in HEPES buffer containing 4 M urea. Soluble and membrane-associated proteins (MF H =HEPES sample; MF U =urea sample) were separated by ultracentrifugation at 100,000 g for 30 min at 4 °C. The supernatant was discarded and the MF H pellet was resuspended in HEPES and washed twice. Finally, the pellet was resuspended at a final chlorophyll concentration of 1 mg chlorophyll per ml and mixed with 85% sucrose in HEPES buffer to reach a final sucrose concentration of 68%. Membranes, containing 200 μg chlorophyll, were loaded below a linear 34–68% SD gradient. All gradients were fractionated after centrifugation at 4 °C, followed by absorbance measurements and immunoblot analyses. The MF U pellet was resuspended and incubated for 30 min in HEPES buffer containing 4 M urea. Afterwards, the sample was pelleted and washed twice with HEPES buffer as described before. Subsequent sample preparation and analysis were performed as described, except that 3 μg of the purified recombinant IM30 was added to the sample before adjusting the sample to 68% sucrose. Liposome preparation The lipids DGDG, DOPC (dioleoylphosphatidylcholine), DOPG (dioleoylphosphatidylglycerol) and MGDG were purchased from Avanti Polar Lipids, Inc. SQDG was from Larodan Fine Chemicals. The fluorescence dyes NBD-PE (1,2-distearoyl- sn -glycero-3-phosphoethanolamine-N-(7-nitro-2-1,3-benzoxadiazol-4-yl)) and LissRhodPE (Lissamin Rhodamin PE; 1,2-Dioleoyl- sn -glycero-3-phosphoethanolamin- N -(lissamin-rhodamin-B-sulfonyl) were purchased from Avanti Polar Lipids, Inc. For liposome preparation, lipids were dissolved in organic solvents. The organic solvent was removed under a gentle stream of nitrogen gas and final traces of the solvent were removed by vacuum desiccation overnight. The dried lipid films were hydrated in HEPES buffer, resulting in formation of multi-lamellar liposomes. Unilamellar liposomes were prepared by five cycles of freezing and thawing, followed by 15 times extrusion through a 100-nm filter, using an extruder from Avanti Polar Lipids, Inc. SD gradient analyses of IM30 binding to liposomes A measure of 0.4 mg of the individual lipids or of lipid mixtures (50%:50%, w/w) were dissolved in organic solvent together with NBD-PE (1:500 molar ratio) before liposome preparation. After preparation of unilamellar liposomes, the size of the liposomes was adjusted to 50 nm by extrusion. Three-micrograms of protein were added, and the samples were incubated for 10 min prior to loading the sample onto the SD. For flotation analyses, 5–50% SD gradients were run at 25 °C and analysed as mentioned above. Laurdan fluorescence measurements To determine the concentration of the non-bilayer forming lipid MGDG tolerated in mixed liposomes, MGDG was mixed with DOPG in increasing concentrations, in 10% increments (compare Supplementary Fig. 7 ). The fluorescence probe Laurdan (6-Dodecanoyl- N , N -dimethyl-2-naphthylamine, from Sigma, Taufkirchen, Germany) was added to each sample at a 1:500 molar ratio. The lipid concentration was adjusted to 0.1 mM by addition of HEPES buffer. Laurdan fluorescence emission was monitored on a Horiba Scientific FluoroMax-4 at 25 °C, from 400 to 550 nm after excitation at 350 nm with both the excitation and emission slit-width set at 4 nm. For the experiments shown in Supplementary Fig. 2 , 80% DOPC lipid was mixed with 20% of one of the four thylakoid lipids (w/w). Laurdan was added to each sample at a 1:500 molar ratio. A final sample concentration of 0.1 mM lipid was reached after adding 2.5 μM IM30 or an equal volume of HEPES buffer before the measurement. Generalized polarization (GP), a measure for membrane fluidity/structure, was calculated as described in Parasassi et al . [52] . Liposome aggregation monitored by light scattering As addition of divalent cations to thylakoid lipids results in membrane aggregation and an increased turbidity of the lipid solution [36] , [37] , we have determined whether addition of IM30 influences the turbidity. Liposomes containing 60% MGDG and 40% DOPG were prepared as described. The final lipid concentration was 0.1 mM for each sample. 2.5 μM IM30 was added to each sample or solely HEPES buffer (control). Cations were added to the desired concentration (Mg 2+ , Ca 2+ : 0–30 mM; Na + . K + : 0–250 mM), the sample was gently mixed by pipetting. After incubation for 5 min at 25 °C, changes in turbidity were monitored at 600 nm. Liposome content release ANTS (8-aminonaphtalene-1,3,6-trisulfonic acid) and DPX ( p -xylene- bis -pyridinium bromide) were purchased from Life Technologies. To determine whether release of soluble liposome content might be induced by addition of Mg 2+ or IM30 (or both), release of soluble liposome content was monitored following the procedure described in refs 53 , 54 . LissRhodPE was added at a molar ratio of 1:550 to the lipid mixture (MGDG/DOPG (60:40 (w/w)) before evaporation of the organic solvent. The dried lipid film was resuspended in HEPES buffer containing 12.5 mM ANTS (fluorescent donor) and 45 mM DPX (quencher), and 100 nm unilamellar liposomes were prepared by extrusion. Free fluorophore and quencher were removed by gel filtration using a Sephadex-25 column. The lipid concentration was determined by measuring the LissRhodPE absorbance at 568 nm using the extinction coefficient ɛ LissRhodPE (88,000 l mol −1 cm −1 ). 0.17 mM lipid was used in the final measurements. ANTS fluorescence at 530 nm was monitored at 25 °C after excitation at 360 nm with both the excitation and emission slit-width set at 8 nm. Complete leakage was induced by adding 1% (v/v) Triton X-100 to preformed liposomes. The measurements were performed either in the presence of 3.9 μM IM30 and increasing MgCl 2 concentrations (0–10 mM from a 1 M stock solution), or in the presence of 7.5 mM MgCl 2 and increasing IM30 concentrations (0–3.9 μM from a 15 μM stock solution). The leakage rate was calculated by where I t is the ANTS fluorescence after time t , I t,100% is the maximal ANTS fluorescence determined using the control sample for complete leakage at time t and I t,0% is the ANTS fluorescence of the negative control sample at time t . For the quantification of the leakage rates, the first 100 s of the measurement were fitted by linear regression and the initial slope was calculated. Liposome fusion To determine whether IM30-induced liposome fusion depends on the Mg 2+ concentration, fusion assays were performed and evaluated essentially as described in Meers et al . [55] . 0.8 μM LissRhodPE (FRET-donor) and 0.8 μM NBD-PE (FRET-acceptor) were added to 0.1 mM lipids (60% MGDG, 40% DOPG, w/w) and liposomes were prepared as described. Unlabelled liposomes were produced without the fluorescence probes. Labelled and unlabelled liposomes were mixed at a ratio of 1:9 (v/v) to achieve a final lipid concentration of 0.1 mM for each sample. The measurements were performed either in the presence of 2.5 μM IM30 and increasing MgCl 2 concentrations (0–10 mM) or in the presence of 7.5 mM MgCl 2 and increasing IM30 concentrations (0–2.5 μM). NBD-PE fluorescence emission at 535 nm was followed at 25 °C after excitation at 460 nm, with both the excitation and emission slit-width set at 5 nm. To determine the FRET value for 100% fusion, 0.1 mM mock-fused liposomes were prepared, containing 0.08 μM of both, LissRhodPE and NBD-PE [55] . Nanoparticle tracking analysis Unilamellar liposomes (60/40 MGDGD/DOPG with LissRhod-PE added in a molar ratio of 500:1) of 100 nm size were prepared by extrusion in HEPES buffer, as described. A 100-μl reaction stock, containing 0.15 mM lipid, 1.3 μM IM30 and 7.5 mM MgCl 2 , was prepared. After the desired reaction time, 10 μl from this stock was diluted 1:2,000 into buffer in order to stop the reaction. Particle size distributions were determined by single-particle tracking based on the fluorescence signal (NanoSight LM10, Malvern Instruments, λ ex =532 nm, emission filter 565 nm long-pass, 25 °C). For each sample, 30 s of particle movement were recorded ten times and the size distribution was calculated as the average from the distribution for each single measurement, as calculated by the software (NTA2.3). The final distribution for each sample was normalized with respect to the derived particle concentration. Membrane destabilization followed by NBD fluorescence For measuring IM30-induced membrane destabilization, unilamellar liposomes (60%/40% MGDG/DOPG (w/w) with NBD-PE added in a molar ration of 500:1) were prepared as described. The measurement was performed at 10 °C using a lipid concentration of 0.15 mM. The time-resolved NBD-PE fluorescence was recorded at 535 nm after excitation at 460 nm with the slit-width set to 4 nm. After 120 s, sodium dithionite was added from a 1 M stock to a final concentration of 10 mM. After 300 s, IM30 and/or MgCl 2 were added, respectively, and fluorescence was recorded for further 300 s. As positive control, 1% (v/v) Triton X-100 was added before the measurement to dissolve the membranes. All samples were incubated at 10 °C for 5 min before the measurement. Transmission electron microscopy Preparation of samples for cryo-electron microscopy was conducted using 3.5 μl of sample on C-flat CF-2/2-2C-T holey carbon grids (Protochips Inc.). Before sample preparation, the grids were washed for 45 min in chloroform, rinsed in acetone, dried and finally glow discharged for 30 s at 25 mA in an Emitech K100X glow discharge system (Quorum Technologies Ltd). Samples containing MgCl 2 were vitrified for either 1 or 30 min after the addition of MgCl 2 to the respective samples. Images were taken on a FEI Tecnai 12 transmission electron microscope (acceleration voltage: 120 kV; Cs: 6.3; nominal magnification: × 71,540; nominal underfocus: 1–3 μm) equipped with a TVIPS TemCam-F416 4K CCD camera. A low-resolution structure of IM30 rings was provided by 3D electron microscopy of negatively stained recombinant protein, as described in Saur et al . [56] For negative staining, continuous carbon EM grids (Protochips Inc.) were negatively glow discharged at 25 mA for 30 s in an Emitech K100X glow discharge system (Quorum Technologies Ltd). Five microlitres of the sample were placed onto an EM grid and incubated for 1 min. Subsequently, the sample was washed three times with water by dragging three 20 μl water drops across a strip of Parafilm (Bemis Europe). After side-blotting the grid with Whatman filter paper No. 4 (GE Healthcare Europe GmbH), a 5-μl droplet of 2% uranyl formate was taken up with the grid and side-blotted after 1 min. Subsequently, the sample was imaged in a FEI Tecnai 12 microscope (120 kV, Cs=6.3, nominal magnification= × 71,540; nominal underfocus: 0.5–1.5 μm; FEI Company) equipped with a TVIPS TemCam-F416 4K CCD camera (TVIPS GmbH). Particles were manually selected from the micrographs and classified in IMAGIC5 (Image Science Software GmbH) using reference-free alignment, multivariate statistical analysis and multiple reference alignment. The heterogeneous data set was initially separated using simulated models of different ring sizes—which were built using stacked 2D class averages—as references in the multirefine procedure of EMAN1.9 (ref. 57 ). For further separation, one ring monomer of the resulting 3D reconstructions was excised and used in differently sized simulated rings as references. The depicted reconstruction has been calculated in a total of 120 iterations in the EMAN1.9 and IMAGIC5 software packages and symmetrized with a 18-fold cylindrical point-group symmetry. Its resolution is approximately 25 Å according to the 0.5 criterion. SFG spectroscopy SFG spectra of IM30 interacting with lipid monolayers were collected at room temperature after 30 min incubation time of 12.6 μM IM30 in HEPES (pH 7.2, 10 mM) with a binary lipid monolayer (60% DOPG, 40% MGDG) in a 25-ml Teflon-coated metal trough. The lipid monolayer was prepared by spreading the lipid mixture, which was dissolved in chloroform, onto a HEPES-buffered solution to a final surface pressure of 14 mN m −1 . The surface pressure was measured with a DeltaPi instrument (Kibron inc.). The protein solution was injected beneath the lipid monolayer. The SFG setup has been described previously in detail [58] . Briefly, a 5-mJ pulse centred at ∼ 800 nm was generated by a Ti:sapphire fs-laser oscillator (MaiTai, Spectra-Physics) and a regenerative amplifier (SpitFire Pro, Spectra-Physics), which was pumped by a Nd:YLF laser (EMPower, Spectra-Physics). One part of the amplifier output (0.5 mJ) was branched off and spectrally narrowed by an etalon to generate a narrow band pulse ( ∼ 15 cm −1 ). The second part was used to generate a tunable infrared pulse with an optical parametric amplifier system (TOPAS, Light Conversion). To generate the SFG signal, the infrared and visible beams were spatially and temporally overlapped on the sample. The SFG signal was then focused onto an emCCD camera (Newton, Andor). The sample stage was purged with nitrogen until the relative humidity was lower than 10%. The SFG spectra were normalized using a reference spectrum obtained from silver in PPP polarization (P-polarized SFG, visible and infrared radiation, respectively). The energy scale of the spectra was calibrated by using the ∼ 1,737 cm −1 lipid C=O stretch peak [59] . VSFG spectra calculations The VSFG spectra are calculated using the formalism described in ref. 60 . The IM30 monomer structural model for which the spectra are calculated is obtained from Bultema et al . [61] The intramolecular hydrogen bonds and contacts with surrounding water were calculated using a short, 1 ns molecular dynamics (MD) simulation in the software package GROMACS. In this simulation, the modelled IM30 monomer used for the VSFG spectra simulation was hydrated and relaxed using the TIP3 and CHARMM27 force fields for the waters and the protein, respectively. We construct the amide-I excitonic Hamiltonian for the amide backbone modes that generate the experimentally observed VSFG response from the protein conformation. The couplings between the nearest neighbour amide-I modes are obtained using an ab initio 6-31G +(d) B3LYP-calculated map that gives the coupling as a function of the dihedral angle between the amide groups [62] . The other couplings, between non-nearest neighbour amide-I modes, are estimated using the transition dipole coupling model [63] . The hydrogen bond-induced frequency shifts of the local amide-I modes are calculated using the empirical model described in Roeters et al . [60] We diagonalize the Hamiltonian to obtain the delocalized amide-I normal modes (eigen vectors) and frequencies (eigen values) of the system. After calculating the infrared and Raman response of the normal modes, we determine the VSFG hyperpolarizability by taking the tensor product of the two responses. To account for homogeneous broadening, we convolute the result with a Lorentzian line shape. The response is transformed from the molecular frame to the lab frame by averaging the Euler transformation between the two frames over the orientational distribution of the molecules [64] , [65] , which gives the nonlinear susceptibility . We calculate the C=O stretch VSFG response of the lipids with the same formalism, except that no hydrogen-bond shifts are taken into account, as this gives the most accurate results for the calculation of the SSP and SPS VSFG spectra of a pure 60/40% DOPG/MGDG binary lipid monolayer. The total VSFG intensity is proportional to the modulus square of the weighted sum of the lipid and protein response: with PLR being the protein oscillator-to-lipid oscillator ratio near the interface. Thus, the calculated VSFG response is dependent on the orientation and magnitude of the transition dipole moment μ and Raman polarizability tensor α of the local modes of the system, the protein and lipid orientation distribution, the line widths of the Lorentzians of the protein and lipid normal modes, Γ protein amide-I and Γ lipid ester-C=O , the overall frequency offsets for the amide-I and ester C=O stretch modes, ν 0 , protein amide-I and ν 0 , lipid ester-C=O , and on the PLR. To fit the model to the experimental data, we include an overall scale factor for each polarization combination. We estimated the magnitude of the transition-dipole moment | μ | of the MGDG lipid to be 0.39 D by measuring the FTIR spectrum of the similar lipid DOPC and used the previously determined transition dipole moment of the amide-I mode (0.37 D) [66] . We determine the orientations of the local-mode μ s based on the transition charges in the amide plane [66] , [67] and the orientations and magnitudes of the α s based on previous work of Tsuboi et al . [68] The orientation distribution of the ester groups in the MGDG/PG lipid monolayer layer was determined from a published MD trajectory [69] . IM30 was treated as a cylindrical protein that most likely has an azimuthally isotropic distribution at the lipid monolayer, so that its VSFG response is only dependent on the Euler angle θ (the angle between the helical axis and the surface normal of the monolayer), as the other two Euler angles φ and ψ average out in the orientation-distribution averaged Euler transformation from the molecular frame to the lab frame. By least-squares fitting the calculated VSFG spectra of IM30 and the lipid monolayer to the experimental SSP and SPS data, we determined the optimal values of Γ protein amide-I , Γ lipid ester-C=O , ν 0 , protein amide-I and ν 0 , lipid ester-C=O . Assuming that at most a single full protein monolayer coverage is possible, the PLR has an upper limit as a function of θ (see Supplementary Fig. 5 ). We estimate this limit from the surface density of lipid monolayers, and assume a cylindrical shape for IM30. If there is less than a full monolayer protein coverage (for example, due to an empty space in the middle of a ring structure comprised of IM30 molecules), the PLR decreases, so PLR values below the line in Supplementary Fig. 5b are also physically plausible. Only calculated SSP spectra for θ 3° and SPS spectra for θ 15° match the experimental spectra well (see Fig. 5c and Supplementary Fig. 5 ). The observation that only small values of θ IM30 are consistent with the experimental data is because, for both the SSP and the SPS polarization combination, the VSFG intensity at 1,650 cm −1 (helical secondary structure of IM30) decreases monotonously for increasing values of θ . Therefore, the spectra can only be fitted well for small values of θ , for which the protein signal is relatively strong; only for the small angles, the inferred PLR is smaller than the physically plausible upper limit of 10. We determined the orientation distribution solely based on the spectral line shapes of the individual polarization combinations, and not from the intensity ratios between the polarization combinations (analogous to the approach described in Roeters et al . [60] ). This approach does not require an accurate description of the reflections at the interface, via the so-called the Fresnel factors [64] , [70] . Therefore, the uncertainty in Fresnel factors (dependent on the intrinsically uncertain interfacial refractive index) does not influence the derived orientation distribution. How to cite this article: Hennig, R. et al . IM30 triggers membrane fusion in cyanobacteria and chloroplasts. Nat. Commun. 6:7018 doi: 10.1038/ncomms8018 (2015).